Photon-mediated interaction between distant quantum dot circuits Engineering the interaction between light and matter is an important goal in the emerging field of quantum opto-electronics. Thanks to the use of cavity quantum electrodynamics architectures, one can envision a fully hybrid multiplexing of quantum conductors. Here we use such an architecture to couple two quantum dot circuits. Our quantum dots are separated by 200 times their own size, with no direct tunnel and electrostatic couplings between them. We demonstrate their interaction, mediated by the cavity photons. This could be used to scale up quantum bit architectures based on quantum dot circuits or simulate on-chip phonon-mediated interactions between strongly correlated electrons. Cavity QED allows one to study the interaction between light and matter at the most elementary level, for instance, by using Rydberg atoms coupled to cavity photons [1] . Recently, it has become possible to perform similar experiments on-chip, by using artificial two-level systems made from superconducting circuits instead of atoms [2] . This circuit–QED offers unexplored potentialities, as other degrees of freedom than those of superconducting circuits could be used [3] , [4] , [5] , [6] , [7] , [8] , [9] , [10] , and in particular, those of quantum dots [11] , [12] , [13] , [14] . Such a hybrid circuit–QED would allow one to study a large variety of situations not accessible with standard cavity QED, owing to the versatility of nanofabricated circuits [7] , [15] . A highly desired functionality required for the use of quantum dots for quantum information processing is the controlled coupling between distant quantum dots. This would allow one to scale up the existing spin quantum bit architectures [16] , [17] , [18] . Among the possible methods for coupling quantum dots [16] , [19] , [20] , the use of photons is particularly attractive because they can mediate a coherent interaction over macroscopic distances [1] , [21] , [22] . Recently, the coupling of single quantum dot circuits to microwave photons has been demonstrated. So far, this architecture has been used to directly measure the electron–photon coupling strength [11] , [12] , [14] or to read-out capacitively a spin quantum bit [13] . Here, we demonstrate a distant interaction by embedding two quantum dot circuits in a microwave cavity. Our quantum dots are separated by 200 times their own size, with no direct tunnel and/or electrostatic coupling. We use one of the two dots as a detector or perform a joint read-out of the two quantum dots with the microwave cavity in order to probe the distant interaction. The spectroscopy of the detector dot is shown to display a dispersion as well as crossings of charge states as a function of its own gate and that of the other distant dot. The joint read-out allows us to probe in a complementary fashion the distant coupling scheme through the phase of the microwave signal. Sample geometry The device presented here is shown in Fig. 1a (see Methods ). The two quantum dots, made using different and well separated single-wall carbon nanotubes, are first studied using the traditional transport spectroscopy. The colourscale plots of the differential conductance of dot 1 (QD1) and dot 2 (QD2) as a function of their gate and source-drain bias are represented in Fig. 1d , respectively. For QD1, the conductance is close to 2 e 2 / h and displays modulations with the characteristic checker-board pattern of an electronic Fabry–Perot interferometer [23] . The vertical distance between the bright spots allows us to determine a level spacing of about 7 meV. This corresponds to a length of about 200 nm, which is slightly smaller than the lithographically defined length. The quantum dot 1 can be considered as an open quantum dot. The differential conductance of QD2 is much smaller and peaks only up to 0.03 × 2 e 2 / h . The colourscale plot of its differential conductance displays Coulomb diamonds and excited states characteristic of the Coulomb blockade regime [24] . In particular, one can read off a charging energy of about 12 meV. Another important parameter for both dots is the width Γ 1(2) of their energy levels. From the colourscale plots, one finds, Γ 1 ≈7 meV and Γ 2 ≈1 meV. This shows that the two electronic systems still relax much faster than the characteristic period of the photonic mode, which corresponds to 5.75 GHz 30 μeV as shown in Fig. 1b . 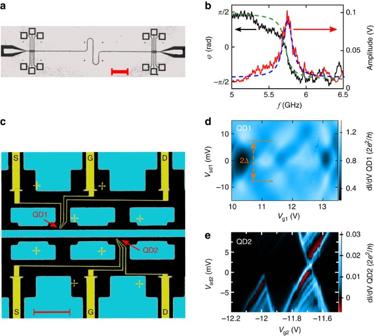Figure 1: The coupling architecture. (a) Optical micrograph of the Al microwave resonator in coplanar waveguide geometry. Four sets of three DC lines allow to contact up to four QDs inside the cavity. The bar is 1 mm. (b) Transmitted amplitude (red curve) and phase (black curve) of the microwave field versus frequency, givingf0=5.75 GHz andQ≈40. (c) False colours optical micrograph showing the two quantum dots structures inside the microwave cavity. Aluminium elements of the resonator are represented in blue (transmission line and ground plane). The Pd DC lines contacting the carbon nanotubes (not visible here), are represented in yellow. The two QDs are separated by 80 μm and are designed by the standard source-drain and side gate geometry. The bar is 50 μm. (d) Colour scale plot of QD1 differential conductance in units of 2e2/hin the gate voltageVg1-bias voltageVsd1plane. The spectroscopy shows a Fabry–Perot behaviour with a level spacing of 7 meV, corresponding to a 200 nm long quantum dot. (e) Colour scale plot of QD2 differential conductance in units of 2e2/hin the gate voltageVg2-bias voltageVsd2plane. The spectroscopy shows a Coulomb diamond with excited states. Figure 1: The coupling architecture. ( a ) Optical micrograph of the Al microwave resonator in coplanar waveguide geometry. Four sets of three DC lines allow to contact up to four QDs inside the cavity. The bar is 1 mm. ( b ) Transmitted amplitude (red curve) and phase (black curve) of the microwave field versus frequency, giving f 0 =5.75 GHz and Q ≈40. ( c ) False colours optical micrograph showing the two quantum dots structures inside the microwave cavity. Aluminium elements of the resonator are represented in blue (transmission line and ground plane). The Pd DC lines contacting the carbon nanotubes (not visible here), are represented in yellow. The two QDs are separated by 80 μm and are designed by the standard source-drain and side gate geometry. The bar is 50 μm. ( d ) Colour scale plot of QD1 differential conductance in units of 2 e 2 / h in the gate voltage V g1 -bias voltage V sd1 plane. The spectroscopy shows a Fabry–Perot behaviour with a level spacing of 7 meV, corresponding to a 200 nm long quantum dot. ( e ) Colour scale plot of QD2 differential conductance in units of 2 e 2 / h in the gate voltage V g2 -bias voltage V sd2 plane. The spectroscopy shows a Coulomb diamond with excited states. Full size image Calibration of electron–photon coupling for each dot Before going to the main result of the present work, which is the distant interaction between the above described quantum dots, it is essential to calibrate the electron–photon coupling for each dot. In order to do this, we apply a strong, classical, microwave drive to the cavity at the resonance frequency. We first focus on the closed dot that allows us to obtain the highest spectral resolution as it has the smallest coupling rate to its reservoirs. The colourscale plots of the differential conductance of QD2 as a function of V g2 and V sd2 for no microwave power, −45, and −35 dBm at the input of the cavity are presented in Fig. 2a–c , respectively. The microwave field splits dynamically the charge degeneracy line crossing at about V g2 =−11.7 V. This splitting is about 3 meV at −45 dBm and increases up to 10 meV at −35 dBm. One can understand classically the observed phenomenon by using the fact that the dot’s electrons have a relaxation rate to the electrodes, which is about 45 times higher than the microwave frequency of the cavity. The AC field of the resonator modulates the dot’s energy levels with an amplitude λV AC and frequency f 0 . The averaging of this modulation leads to split conductance peaks (dashed lines) at E 0 ± λV AC , as depicted schematically in Fig. 2d . The differential conductance G on ( V g , V sd ) at finite microwave drive can be obtained by assuming that the microwave field only couples to the electronic levels, leading to: , λ characterizing the electron–photon coupling strength, V AC being the amplitude of the AC voltage at the resonator frequency f 0 and G off ( V g , V sd ) being the differential conductance of QD2 with no microwave power. The results of this procedure is shown in Fig. 2e , respectively, for λ =15.5, using the measured data of Fig. 2a . The conductance peak splitting and in particular the peculiar diamond-shaped region emerging at the charge degeneracy point around V g2 =−11.7 V are very well accounted for. Note that not all the features in Fig. 2b are reproduced with our procedure, indicating that some of the excited states might have a different coupling to the photons than the ground state [25] . 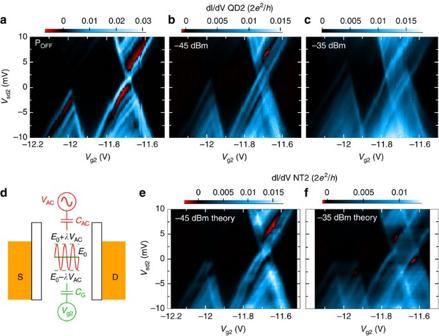Figure 2: Driving quantum dot 2 through the cavity. Influence of the microwave power driving the cavity on QD2 spectroscopy. Differential conductance of QD2 as a function of the gate voltageVg2and the bias voltageVsd2for different powers at the input port of the cavity: (a) no power, (b)Pin=−45 dBm and (c)Pin=−35 dBm. The conductance peaks of the quantum dot split, as emphasized by the formation of a new diamond-shaped region aroundVg2=−11.7 V. (d) Scheme showing the capacitive coupling of the quantum dot electronic levels to the gate electrode (green) and to the resonator (red). The DC gate electrode drives the level energyE0in the quantum dot. The AC field of the resonator modulates the energy levels with an amplitudeλVACand frequencyf0. The averaging of this modulation leads to two split conductance peaks (dashed lines) atE0±λVAC. Simulations of the splitting based on the scheme depicted in (d) and applied to the spectroscopy of (a) withλ=15.5, respectively, forPin=−45 dBm (e) andPin=−35 dBm (f). Figure 2: Driving quantum dot 2 through the cavity. Influence of the microwave power driving the cavity on QD2 spectroscopy. Differential conductance of QD2 as a function of the gate voltage V g2 and the bias voltage V sd2 for different powers at the input port of the cavity: ( a ) no power, ( b ) P in =−45 dBm and ( c ) P in =−35 dBm. The conductance peaks of the quantum dot split, as emphasized by the formation of a new diamond-shaped region around V g2 =−11.7 V. ( d ) Scheme showing the capacitive coupling of the quantum dot electronic levels to the gate electrode (green) and to the resonator (red). The DC gate electrode drives the level energy E 0 in the quantum dot. The AC field of the resonator modulates the energy levels with an amplitude λV AC and frequency f 0 . The averaging of this modulation leads to two split conductance peaks (dashed lines) at E 0 ± λV AC . Simulations of the splitting based on the scheme depicted in ( d ) and applied to the spectroscopy of ( a ) with λ =15.5, respectively, for P in =−45 dBm ( e ) and P in =−35 dBm ( f ). Full size image The specific origin of the conductance peak splitting can be confirmed by studying its dependence as a function of the power of the microwave signal at the input of the cavity, or equivalently the average number of photons stored in the cavity. Although we have used a classical field so far, such a study allows us to determine accurately the electron–photon coupling terms entering into the Anderson–Holstein-like Hamiltonian of the system [11] , , being the total number of electrons in QD1(2) and a ( a † ) being the annihilation (creation) operators for the photons in the cavity at the fundamental frequency. This will allow us below to predict the expected form and magnitude of the interaction between the two dots, which are dominated by single-photon processes. Such a study is shown in Fig. 3a for QD1 and QD2, respectively. The colourscale plot of the differential conductance of the dots as a function the source-drain bias and the input power displays a characteristic funnel shape showing the conductance peak splitting in QD1 and QD2 as the power is increased. According to the picture developed previously, the splitting should scale linearly with the amplitude of the field, or equivalently with the square root of the average number of photons. The latter viewpoint is particularly convenient as it allows us to determine directly the coupling constants of QD1 and QD2 to a single photon, g 1 and g 2 , respectively. Indeed, the splitting Δ 1(2) reads: , where is the average number of photons in the cavity. The dependence of Δ 1(2) as a function of is shown in the inset of Fig. 3a for QD1 and 2, respectively. The linear behaviour observed fully confirms our level driving picture and allows us to determine g 1 =97±22 MHz and g 2 =98±22 MHz. We emphasize again that we obtain them by re-expressing the driving amplitude for each dot using . The uncertainty in the determination of g 1(2) is mainly related to the systematic errors made in the determination of the exact power at the input of our cavity. 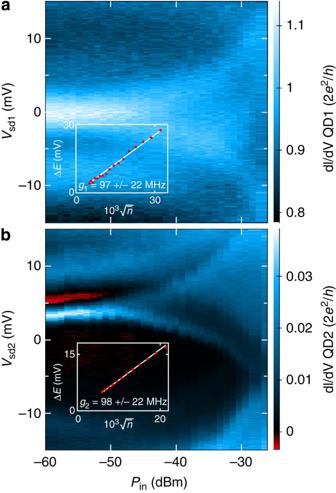Figure 3: Measurement of the electron–photon coupling strength for each dot. Microwave power dependence of conductance peak splitting. (a,b) Colour scale plots of the differential conductance of QD1 (respectively QD2) in the input powerPin-bias voltageVsd1(respectivelyVsd2) plane. Insets: the dependence of the conductance peak separation ΔEversusfor each QD (red dots). The slope of the linear fit (white line) gives the couplingg1(2)between the quantum dot 1(2) and the microwave field as. Figure 3: Measurement of the electron–photon coupling strength for each dot. Microwave power dependence of conductance peak splitting. ( a , b ) Colour scale plots of the differential conductance of QD1 (respectively QD2) in the input power P in -bias voltage V sd1 (respectively V sd2 ) plane. Insets: the dependence of the conductance peak separation Δ E versus for each QD (red dots). The slope of the linear fit (white line) gives the coupling g 1(2) between the quantum dot 1(2) and the microwave field as . Full size image Gate tunable electron–photon coupling We now investigate with greater detail the coupling mechanism between the photons and the electrons on the carbon nanotubes. This section will allow us first to demonstrate interesting ‘toggles’ for the electric control of the electron–photon coupling strength. Importantly, it will allow us to rule out all the spurious DC electrostatic effects, which could hinder the study of the photon-mediated distant interaction between the dots. We focus on QD1 for which electronic interactions can be neglected. The AC response of QD1 can be conveniently predicted with a self-consistent theory of AC transport similar to that of ref. 26 (see Methods ). We measure g 1 for various gate voltages V g1 using the previously described method. The result is presented in Fig. 4b in inset by the filled dots. The value of g 1 displays modulations as V g1 is swept. Strikingly, the change in g 1 is proportional to the linear conductance G 1 of QD1 as shown in Fig. 4b main panel. The value of g 1 increases by almost 100 MHz when the conductance G 1 is increased from 0.3 × 2 e 2 / h to 1.1 × 2 e 2 / h . Such an increase is accounted for by the increase of the quantum capacitance of QD1, which is directly proportional to the conductance G 1 (see Methods ). As shown in Fig. 4b , the sign of the slope of g 1 versus G 1 allows to discriminate between direct coupling between the cavity photons to the dot’s energy level and indirect coupling to the dot’s energy level via the source-drain electrodes. As expected from the efficient screening of the source-drain electrodes, the coupling mechanism is mainly via the source-drain leads, as shown by the positive slope of g 1 versus G 1 (blue continuous line). One can further specify this by comparing the intercept of the blue line with the vertical axis. It corresponds to the geometrical part of the coupling strength of dot 1 as it corresponds to zero conductance. We find 48 MHz. An upper bound of the direct coupling can be obtained by reading off from Fig. 1d the DC side gate lever arm, of about 0.01. This corresponds to only 2 MHz and supports further that the coupling mechanism involves the source and drain leads, and that Fig. 4a best displays the corresponding circuit diagram. Note that this mechanism is only possible at the frequency of the cavity as the source and drain electrodes are DC shunted in order to measure simultaneously the low frequency conductance (below 1 kHz). Therefore, DC potentials on the central conductor of the cavity do not affect the energy levels of QD1 and any change in QD1’s potential does not affect the potential of the central conductor. 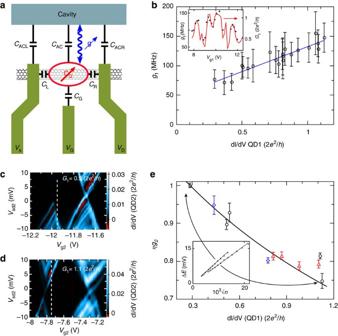Figure 4: Coupling mechanism and tunable coupling strength. (a) Schematics of the coupling mechanism between the quantum dots and the cavity. (b) Variation of the electron–photon coupling strength of QD1, in open dots, as a function of its own linear conductance. The error bars correspond to the systematic error of the linear fitting for the plots in inset ofFig. 3. The solid line is the theory described in theMethodssection. Inset: variations of the electron–photon coupling strength and of the conductance of QD1 as a function ofVg1. (c,d) Transport spectroscopy of QD2 for two different values of the conductance of QD1 (corresponding to two different sets of (Vg2,Vg1) for the same energy level of QD2). (e) Relative variation of the electron–photon coupling strength of QD2 as a function of the linear conductance of QD1. The open circles correspond to a change of the conductance of dot 1 by changing its gate. The open triangles and diamonds correspond to a change of conductance by changing the source-drain bias. The solid black line is the theory. Inset: the dependence of the conductance peak separation ΔEversusfor the two points indicated by the arrows. The error bars correspond to the systematic error of the linear fitting for the plots in the inset ofFig. 3. Figure 4: Coupling mechanism and tunable coupling strength. ( a ) Schematics of the coupling mechanism between the quantum dots and the cavity. ( b ) Variation of the electron–photon coupling strength of QD1, in open dots, as a function of its own linear conductance. The error bars correspond to the systematic error of the linear fitting for the plots in inset of Fig. 3 . The solid line is the theory described in the Methods section. Inset: variations of the electron–photon coupling strength and of the conductance of QD1 as a function of V g1 . ( c , d ) Transport spectroscopy of QD2 for two different values of the conductance of QD1 (corresponding to two different sets of ( V g2 , V g1 ) for the same energy level of QD2). ( e ) Relative variation of the electron–photon coupling strength of QD2 as a function of the linear conductance of QD1. The open circles correspond to a change of the conductance of dot 1 by changing its gate. The open triangles and diamonds correspond to a change of conductance by changing the source-drain bias. The solid black line is the theory. Inset: the dependence of the conductance peak separation Δ E versus for the two points indicated by the arrows. The error bars correspond to the systematic error of the linear fitting for the plots in the inset of Fig. 3 . Full size image Distant coupling between the dots We now probe the coupling between the states of QD1 and those of QD2, which is the central result of this article. We first use QD2 as a detector and measure the evolution of its energy levels via transport spectroscopy as its own gate and the distant gate of QD1 are swept. We present in Fig. 5a the differential conductance of QD2 as a function of V g1 and V g2 for one specific region. Strikingly, the gate of QD1 acts on QD2 even though the direct capacitive coupling is vanishingly small—the wide central conductor has a capacitance to the ground, which is of about 0.7 pF, more than 5 orders of magnitude bigger than the gate capacitances of about 1 aF. Furthermore, as discussed above, the two dots, separated by the central conductor of the cavity, are only AC coupled to the cavity, via the source-drain leads. This strongly points to a distant interaction between the two dots without any direct electrostatic or tunnel coupling. In particular, it is not an electrostatic interaction mediated by a floating gate [27] . 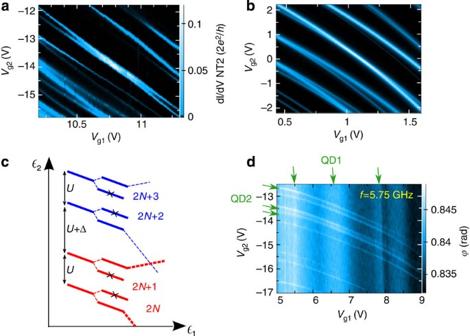Figure 5: Distant coupling between the quantum dots. (a) Colour scale plot of the differential conductance of QD2 versus its own gate voltageVg2and the gate voltageVg1of QD1. The levels of QD2 evolve with different slopes, leading to level crossings. (b) Modelling of the conductance map of QD2 using the form ofpresented in the main text and a simplified equation of motion theory. (c) Diagram of the transport spectroscopy of QD2 versusε2andε1, the energies of QD2 and QD1, respectively. Two orbitals are represented (red and blue levels), separated byU+Δ, with Δ the orbital spacing. The two conductance peaks corresponding to the same orbital are separated by the charging energyU. The interaction between QD1 and QD2 shifts the levels of QD2. They are also split as shown by the dashed lines. The conductance peaks separated by less thanUin the same orbital are forbidden (shown by a cross). Crossings between conductance peaks originating from different orbitals are allowed. The resulting spectroscopic pattern exhibits an alternation of conductance peaks moving away and coming closer, as observed in (a). (d) Joint readout of the two QDs in the phaseφof the transmitted RF signal. Both levels of QD1 and QD2, indicated by green arrows, can be observed and cross. Figure 5: Distant coupling between the quantum dots. ( a ) Colour scale plot of the differential conductance of QD2 versus its own gate voltage V g2 and the gate voltage V g1 of QD1. The levels of QD2 evolve with different slopes, leading to level crossings. ( b ) Modelling of the conductance map of QD2 using the form of presented in the main text and a simplified equation of motion theory. ( c ) Diagram of the transport spectroscopy of QD2 versus ε 2 and ε 1 , the energies of QD2 and QD1, respectively. Two orbitals are represented (red and blue levels), separated by U +Δ, with Δ the orbital spacing. The two conductance peaks corresponding to the same orbital are separated by the charging energy U . The interaction between QD1 and QD2 shifts the levels of QD2. They are also split as shown by the dashed lines. The conductance peaks separated by less than U in the same orbital are forbidden (shown by a cross). Crossings between conductance peaks originating from different orbitals are allowed. The resulting spectroscopic pattern exhibits an alternation of conductance peaks moving away and coming closer, as observed in ( a ). ( d ) Joint readout of the two QDs in the phase φ of the transmitted RF signal. Both levels of QD1 and QD2, indicated by green arrows, can be observed and cross. Full size image Both quantum dots are coupled to the fundamental mode of the cavity. They can a priori be coupled via the virtual exchange of photons in a similar fashion as in atomic physics [1] , [21] , [28] . The equivalent interaction mechanism, found in condensed matter whenever electronic states are coupled to bosonic modes, leads to a polaronic shift of each of the levels of QD1(2): being the number of electrons in QD2(1), respectively [29] , [30] . This shift can be simply found from a Lang–Firsov transformation of the dot’s total Hamiltonian (see Methods ). As QD1 can contain a large number of electrons, Δ 2 polaron can become large, comparable to the energy scales relevant for QD2. This shift therefore survives at our moderately low temperatures even though the essence of this interaction is mainly quantum mechanical. One finds, for example, Δ 2 polaron ≈−1 meV for N 1 ≈10 4 . As shown in Fig. 4 , g 1 and g 2 strongly depend on the gate voltage of QD1 and QD2, respectively. This means that even though N 2(1) are large numbers and do not vary substantially as the gates of each dot are swept, the shift can still evolve thanks to the gate tunability of the g ′s as V g1(2) are varied. We now use with the range of α 1(2) extracted from Fig. 4 . Note that the hierarchy of energy scales here is the same as for phonons in solids, which are usually much slower than the electrons, the electrons being delocalized over many sites. Physically, electrons on QD1 and QD2 shift the electric field corresponding to the cavity photons. The modification of the circuit energy by this effect is twofold. First, as QD2 is coupled to the cavity, the electrons of QD2 directly feel the photonic electric field deformation induced by the electrons of QD1. Second, as the energy of the cavity involves quadratically the photonic electric field, the shift of this electric field by electrons of both QD1 and QD2 produces crossed terms between QD1 and QD2. These two phenomena lead to a global effective interaction between the two dots’ electronic states. In addition to the shift, the coupling of electrons to photons can lead to a splitting of the energy levels in each dot, proportional to the coupling constant of each dot to the photons. This can arise for instance owing to photon-induced K–K’ mixing as predicted recently [25] . The general form of the energy levels of QD2 is therefore , ε 0 being a constant, α 0 characterizing the bare coupling of QD2 to its gate and δ characterizing the magnitude of the splitting. The gate dependence of g 2 implies a variation of the splitting as gate 2 and gate 1 are swept, which explains the crossings of conductance peaks observed in Fig. 5a . As shown in Fig. 5b , we are able to reproduce with a simple modelling all the features observed in Fig. 5a (see Methods ). The values of α 1(2) and N 1 are the three fitting parameters used to produce the main slope in Fig. 5b (see Methods ). The origin of the crossings is sketched schematically in Fig. 5c . The distant coupling can be used to control in a non-local manner the electron–photon coupling strength, as it shifts the energy levels of each dot. We illustrate this fact by studying the evolution of g 2 as a function of G 1 , as shown in Fig. 4e . The open circles are obtained for zero V sd and different gate voltages whereas all the other points are obtained by varying the source-drain bias at constant gate voltage. The systematic variation (roughly linear) of g 2 as a function of G 1 in the two different conditions depicted above shows that it is G 1 and therefore the quantum capacitance of dot 1 that matters for the shift of the energy levels rather than the gate voltage V g1 itself. As a consequence, it further supports our distant coupling mechanism. As shown in Fig. 5a , we can follow the evolution of the energy levels of QD2 in the ( V g2 – V g1 ) plane. We present in Fig. 4c the bias spectroscopy of QD2 along one of the tilted lines of Fig. 5a for two different sets of ( V g2 – V g1 ). The size of the Coulomb diamonds is different for each of the sets of ( V g2 – V g1 ), which are conveniently expressed in terms of G 1 for similar reasons as above for the study of the local control of g 1 . Measuring g 2 along this line gives the open symbols of Fig. 4e . For each of these points, we extract the capacitive lever arm for the dot from the slope of the Coulomb diamonds. This allows us to predict the dependence of g 2 , according to the coupling mechanism described in the Methods section. The resulting theoretical curve is the black solid line, which accounts very well for our measurements of g 2 . As both quantum dots are coupled to the microwave field, one can perform a joint read-out of their state by measuring the phase of the transmitted microwave signal through the cavity. Such a measurement is presented in Fig. 5d . The levels of QD1 and QD2 are clearly observed as tilted narrow and almost vertical shallow stripes, respectively, in the colourscale plot of the phase at 5.75 GHz as a function of V g1 and V g2 . As expected, the levels of QD1 are wider than those of QD2. Their dependance on the distant gate (of QD2 now) is weaker than for QD2. We explain this fact by the smaller number of electrons N 2 in the closed quantum dot QD2. Note that the levels of QD1 and QD2 cross, which means that they are not coherently coupled by the photons as expected because the ‘gammas’ are too large. The origin of the observed interaction relies, however, on the exchange of virtual photons like for the mechanism leading to two quantum bit operations for Rydberg atoms or superconducting quantum bits [1] , [21] , [22] . As the g 1 , g 2 electron–photon couplings are the same as for the transmon-type quantum bits, we can therefore envision to perform SWAP operations as fast as for superconducting quantum bits. This will require converting the coupling to the charge to a coupling to the the spin [5] , [6] and using more isolated quantum dots. Experimental Two single quantum dot circuits are fabricated using two different and well separated single-wall carbon nanotubes connected to normal (Pd) electrodes, inside an Al microwave cavity shown in Fig. 1a (see ref. 11 for details). Both dots share the same antinode of the electric field of the fundamental mode of the resonator, but they are located on opposite sides of the central conductor of the resonator, as shown in Fig. 1c . Their lateral size defined by nanolithography is about 400 nm, which is more than two orders of magnitude below the distance between them, about 80 μm. The characteristics of the resonator are shown in Fig. 1b . The fundamental mode frequency is at 5.75 GHz with a quality factor of about 40, as shown by the peak in the amplitude of the transmitted signal in red line. The phase of the microwave signal, shown in black line, displays the characteristic jump of π at the resonance. The temperature of the experiment is 1.5 K throughout the paper. Modelling of the evolution of the conductance peaks One can model the influence of the level structure depicted in the main text on transport in a Coulomb-blockaded quantum dot as QD2. We present in Fig. 5b the result of such a modelling using a simplified equation of motion theory for the Green’s functions and the Meir–Wingreen formula for the linear conductance [31] . The colourscale plot of Fig. 5b has been obtained using N 1 =10 6 and α 1(2) ≈25 MHz V −1 in the { V g1 , V g2 } region considered here. In particular, the alternation between level crossings and splittings as gate 2 is swept towards negative values is reproduced. This phenomenon can be explained qualitatively by the picture of Fig. 5c . In a quantum dot in the Coulomb blockade regime, a splitting of energy levels in the intrinsic spectrum leads to a separation between conductance peaks corresponding to the same orbital and to crossing of conductance peaks corresponding to different orbital levels. Electron–photon coupling mechanism The electrostatics of the dots allows us to determine the level energy at the mean-field level [26] : where N is the average number of charge on the island, ε d is the bare dot energy and E C = e 2 /(2 C Σ ) is the charging energy. The other important terms in the above expression are: α AC the direct cavity–dot capacitive coupling, α L,R the L, R capacitances of the source-drain electrodes and is the source(drain) lead—cavity capacitive coupling that we assume to be the same for source and drain here (symmetric coupling). The self-consistent equation that governs the number of charges on the dot is , with f the Fermi function, μ ec the electrochemical potential of the leads and the spectral density of the dot. The electrochemical potential of the dot is changed via the AC drive V AC of the cavity as . From the above equations, one can derive . The electron–photon coupling then is obtained by the derivative of the dot energy level with respect to the fluctuating potential of the resonator: The charge susceptibility ∂ N /∂ ε d of the dot is the opposite of the quantum capacitance C Q of the dot in the non-interacting limit ((∂ N /∂ ε d )=− C Q / e 2 ) and is proportional to the linear conductance G of the dot [26] . If the dot is directly coupled to the cavity, the above expression shows a negative slope as a function of G whereas if the dot is indirectly coupled via the leads, the above expression shows a positive slope, which arises from the sum rule α L + α R <1. This allows us to plot the blue line of Fig. 4b and to conclude that our dots are coupled to the cavity photons via the dot’s source-drain leads. Distant coupling and Lang–Firsov transformation We reproduce here the Lang–Firsov transformation, which allows us to derive the interaction between the distant dots. We first consider the Anderson–Holstein Hamiltonian of the main text: d corresponds to the different dots. We assume g d dependent on the dot d as the dots are different and located in different positions. The operator H int accounts for the electronic interaction on each dot. We follow ref. 29 and use the unitary transformation for an operator A : with Using the identity: we get: The second term contains two quadratic terms and one bilinear term in the number of electrons occupying each dot. While the first can be absorbed in the interaction term of Hamiltonian of each dot, the bilinear term can be factorized in each orbital part of the Hamiltonian, leading to the expression used in the main text for the polaronic shift. This leads to the distant coupling of the main text. Note that, contrarily to transport where only the states close to Fermi energy matter, it is the total charge that is coupled to the electromagnetic field (the sum goes over all occupied states). This can lead to a very large shift of the levels of each dot provided the distant dot has a high enough charge density. In addition, contrarily to its atomic physics counterpart, the above expression is non-perturbative and is exact when the dot–lead coupling is zero. Using the above equation, we get: This can be further simplified in the continuum limit as: where for QD1. By defining , the implicit equation for { V g2 , V g1 } reads: This is the most important part of the equation of the main text and controls the dispersion of the energy levels of dot 2. As g 1 ( V g1 ) is an integral over all the occupied energy levels, its variations are smooth and roughly linear over a large gate voltage scale. The variations of g 2 ( V g2 ) can be more pronounced and can lead in general to a nonlinear dispersion of the energy levels in the { V g2 , V g1 } plane, as observed in the joint read-out of Fig. 5d . Using the values given in the maintext, we are able to reproduce the observed general slope of the energy levels of QD2 in the { V g2 , V g1 } plane. Note that the above analysis, carried out for a single mode of the electromagnetic field, can be straightforwardly extended to the multimode case. As the coupling mechanism demonstrated here is non-resonant, essentially all the modes within the line width of the energy levels can contribute [30] . This can reduce the number of electrons needed to explain our data by a factor of 100–300. How to cite this article: Delbecq, M.R. et al . Photon-mediated interaction between distant quantum dot circuits. Nat. Commun. 4:1400 doi: 10.1038/ncomms2407 (2013).